Specific adaptation ofUstilaginoidea virensin occupying host florets revealed by comparative and functional genomics Ustilaginoidea virens (Cooke) Takah is an ascomycetous fungus that causes rice false smut, a devastating emerging disease worldwide. Here we report a 39.4 Mb draft genome sequence of U. virens that encodes 8,426 predicted genes. The genome has ~25% repetitive sequences that have been affected by repeat-induced point mutations. Evolutionarily, U. virens is close to the entomopathogenic Metarhizium spp., suggesting potential host jumping across kingdoms. U. virens possesses reduced gene inventories for polysaccharide degradation, nutrient uptake and secondary metabolism, which may result from adaptations to the specific floret infection and biotrophic lifestyles. Consistent with their potential roles in pathogenicity, genes for secreted proteins and secondary metabolism and the pathogen–host interaction database genes are highly enriched in the transcriptome during early infection. We further show that 18 candidate effectors can suppress plant hypersensitive responses. Together, our analyses offer new insights into molecular mechanisms of evolution, biotrophy and pathogenesis of U. virens . Rice false smut (RFS) caused by the pathogenic ascomycete fungus Ustilaginoidea virens (Cooke) Takah (teleomorph: Villosiclava virens ) was first reported from Tirunelveli district of Tamil Nadu State of India in the 1870s [1] , [2] . RFS was once categorized as a minor disease with sporadic occurrence in rice-growing areas. However, it has recently become one of the most devastating grain diseases in the majority of rice-growing areas of the world due to extensive planting of high-yielding cultivars and hybrids, overuse of chemical fertilizers and an apparent change in global and regional climates [3] , [4] , [5] . In particular, RFS has been estimated to occur in one third of the rice cultivation areas in China [5] . RFS has an intriguing disease cycle. U. virens initiates infection through rice floral organs producing white hyphae, and then develops powdery dark green chlamydospore balls in spikelets during the late phase of infection [6] ( Fig. 1 ). As diurnal temperatures fluctuate more in late autumn, sclerotia appear on the surface of spore balls [6] . A key characteristic of RFS is that the pathogen produces two types of mycotoxins, ustiloxins and ustilaginoidins. Ustiloxins are antimitotic cyclic depsipeptides with a 13-membered core structure [7] . Ustiloxins inhibit cell division, especially by inhibiting microtubule assembly and cell skeleton formation [8] . Ustilaginoidins are bi(naphtho-γ-pyrone) derivatives, which exhibit weak antitumor cytotoxicity to human epidermoid carcinoma [9] , [10] . RFS thus not only results in severe yield losses in rice [4] but also contaminates rice grain and straw to potentially cause human or animal poisoning [11] . Many previous studies have focused on isolation and characterization of ustiloxins and ustilaginoidins, but the pathways and genes responsible for their biosynthesis remain largely unknown [12] . 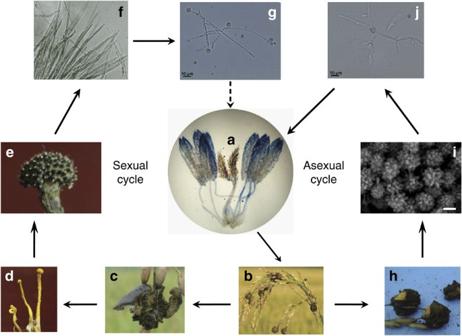Figure 1: Major stages in the infection cycle ofUstilaginoidea virens. (a) Stamen filaments in the florets infected byU. virens. Hyphae were stained with trypan blue to show primary infection sites. (b) False smut balls formed in the rice spikelets. (c) Sclerotia formed on the surface of spore balls. (d) Stroma produced by a germinating sclerotium. (e) Ascocarp formed on the stroma. (f) Asci. (g) Ascospore germination, Scale bar, 10 μm. (h) Spore balls. (i) Chlamydospores under scanning electron microscopy. Scale bar, 3 μm. (j) Chlamydospore germination. Scale bar, 10 μm. Figure 1: Major stages in the infection cycle of Ustilaginoidea virens . ( a ) Stamen filaments in the florets infected by U. virens . Hyphae were stained with trypan blue to show primary infection sites. ( b ) False smut balls formed in the rice spikelets. ( c ) Sclerotia formed on the surface of spore balls. ( d ) Stroma produced by a germinating sclerotium. ( e ) Ascocarp formed on the stroma. ( f ) Asci. ( g ) Ascospore germination, Scale bar, 10 μm. ( h ) Spore balls. ( i ) Chlamydospores under scanning electron microscopy. Scale bar, 3 μm. ( j ) Chlamydospore germination. Scale bar, 10 μm. Full size image U. virens produces both sexual (ascospores) and asexual (chlamydospores) stages in its life cycle ( Fig. 1 ), and thick-walled chlamydospores can survive up to 4 months in the field with sclerotia presumed to survive much longer [13] . Sclerotia on or under soil surface can germinate and form fruiting bodies, and ascospores that contribute to primary infections are then produced after mating and meiosis ( Fig. 1 ) [14] . Some rice weeds and grass species may act as alternative hosts for the pathogen and may be important sources of inoculum between seasons [15] . Previous results suggested that the fungus is both seed borne and soil borne, and can invade seedlings even if infection symptoms are not observed until the flowering stage in rice [16] . However, our knowledge of the disease cycle and infection processes of U. virens is incomplete and sometimes contradictory [5] . The infection process of U. virens was recently investigated through extensive histological examinations [17] . U. virens hyphae enter floral organs primarily at upper parts of the stamen filaments between the ovary and lodicules [17] . U. virens occasionally infects the stigma and lodicules, but is not known to infect the ovaries. Primarily, the pathogen hyphae extend into the central vascular tissues without penetrating rice cell walls directly [17] . Therefore, the pathogen is considered to be a biotrophic parasite [17] . U. virens is the only member of the tribe Ustilaginoideae of the family Clavicipitaceae with a known sexual state, which is rarely observed in nature [13] . Its teleomorph was originally classified as Claviceps virens Sakurai ex Nakata and has been recently re-categorized as Villosiclava virens since it is morphologically distinct from Claviceps [1] . The Clavicipitaceae family consists of 43 genera such as Claviceps , Cordyceps , Epichiloe , Metarhizium and Ustilaginoidea , which include pathogens across animal, plant and fungal kingdoms. Such a broad host range makes this family unique for exploring evolution and host adaptation [18] . It has been speculated that the tribe Ustilaginoideae may have a different origin from other clavicipitaceous fungi [19] . This project takes genomic approaches to dissect molecular mechanisms of RFS for development of effective disease management strategies. Our analyses provide soild phylogenetic placement for U. virens to be closely related to the entomopathogenic Metarhizium spp., Genomic content supports a specific adaptation of this pathogen in occupying host florets, which are rich in sugar content but deficient in cellulose, pectin and other cell wall materials. Genome analyses facilitate the isolation and characterization of genes and regulatory mechanisms that control mycotoxin production. The in planta upregulation of candidate effectors, genes involved in secondary metabolite biosynthesis, as well as the pathogen–host interaction database (PHI-base) [20] genes suggests a list of candidate virulence factors that may play important roles in pathogenicity. Overall, this genome project establishes foundation for the rice Ustilaginoidea pathosystem as a primary target for elucidating the interaction between hosts and biotrophic fungal pathogens. Genome assembly with lower gene density The genome of the U. virens strain UV-8b was assembled from sequencing data generated by Illumina and 454 sequencing technologies ( Supplementary Table 1 ). Data from 454 sequencing were assembled into contigs using the Newbler assembler. 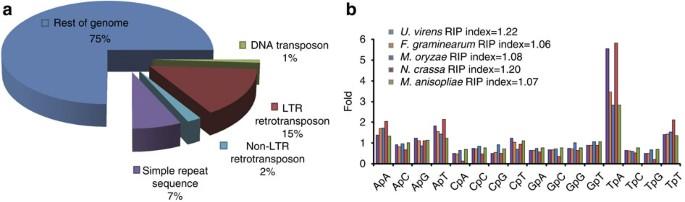Figure 2: Repetitive sequences have been affected by repeat-induced point mutations inU. virens. (a) The proportion (%) of different types of repetitive sequences in theU. virensUV-8b genome. (b) Estimation of RIP for five sequenced ascomycete genomes. Average RIP indices inU. virens, F. graminearum, M. oryzae, N. crassaandM. anisopliaeand the ratio of each type of di-nucleotide (ratio of frequency in repetitive elements to that in non-TEs) in different fungal genomes are shown. Subsequently, these contigs were used as single ends and combined with trimmed paired-end Illumina data for assembly with ABySS [21] , resulting in longer sequences with a total assembly size of 38.8 Mb and an N50 contig length of about 29.3 kb ( Supplementary Table 2 ). Contigs were further linked with SSPACE scaffolder [22] into 449 scaffolds (>2 kb) with an N50 length of 533.6 kb and a total assembly size of 39.4 Mb ( Table 1 , Supplementary Table 2 ) that accounts for 97.5% of the total genome size (~40.4 Mb) estimated by JELLYFISH [23] . High consistency between 454 and Illumina data sets and depth distribution analyses confirm the high quality of the final assembly ( Supplementary Fig. 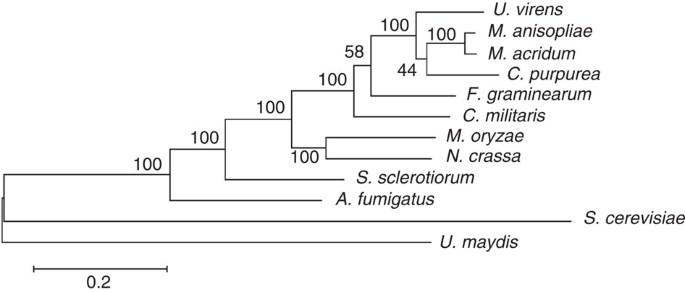Figure 3: Phylogenetic analyses for evolutionary relationships among different fungi. The fungi areU. virens, C. purpurea, M. anisopliae, M. acridum, C. militaris, M. oryzae, F. graminearum, N. crassa, A. fumigatus, S. cerevisiae, S. sclerotiorumandU. maydis. A maximum likelihood phylogenetic tree constructed based on derived protein sequences of 21 single-copy genes common to these 12 fungal genomes that were identified from a set of 74 single-copy orthologous genes across the Kingdom Fungi showing evolutionary relationships among these fungi. 1 , Supplementary Table 3 , Supplementary Note 1 ). 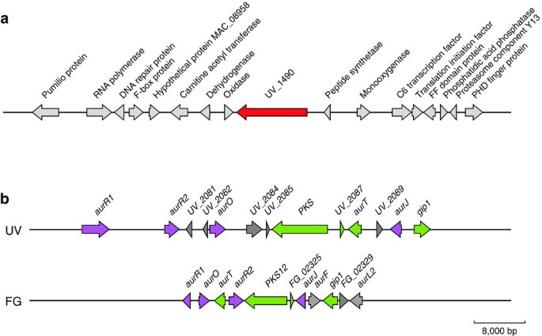Figure 4: Putative NRPS and PKS gene clusters for ustiloxin and ustilaginoidin biosynthetic pathways. (a) The putative NRPS gene (central long red arrow) cluster for ustiloxin biosynthesis. UV_1490 containing three adenylation domains may be responsible for the biosynthesis of the core structure of ustiloxins. The NRPS gene is clustered around genes encoding dehydrogenase, oxidase, monooxygenase and transcription factor that may be involved in the modification of secondary metabolites. (b) Comparison between the putative PKS gene cluster for ustilaginoidin biosynthesis inU. virens(upper) and the aurofusarin biosynthesis gene cluster inF. graminearum(bottom). TheUV_2086(PKS),UV_2087,aurTandgip1genes (green) inU. virenswere identified by BLASTing against the aurofusarin biosynthesis genes while other genes (purple) were predicted via Pfam domain search. TheaurFandaurL2genes (grey) in the aurofusarin biosynthesis gene cluster inF. graminearumare absent inU. virensgenome. Furthermore, all RNA-seq reads were assembled into 17,168 contigs longer than 300 bp, and 99.2% of that are aligned with the genomic sequence, implying high coverage of coding regions in the assembly ( Supplementary Table 4 ). Table 1 Genome features of U. virens UV-8b. Full size table A total of 8,426 protein-coding genes were predicted from the genome assembly, 8,243 of which were supported by the RNA-seq data. The coding regions from the predicted genes constitute 32.7% of the genome with an average gene density of 214 genes per 1 Mb, which is fewer than most of other sequenced ascomycetes [24] , [25] . The average 1,627 bp gene length includes an average 1,414 bp of coding region and 213 bp of non-coding region ( Table 1 ). The GC contents of the genome, coding sequences and repetitive elements are 49.96, 58.42 and 39.77%, respectively. A total of 204 tRNA genes were predicted from the assembly ( Table 1 ). 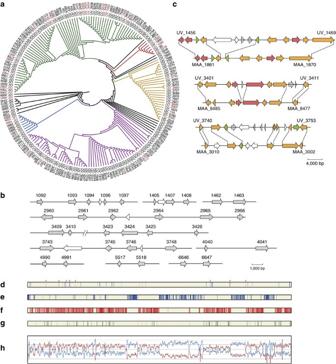Figure 5: Genes and gene clusters encoding putative effectors and their locations in relation to repetitive sequences in theU. virensgenome. (a) A phylogenetic tree of 193 putative effectors indicates that most effectors are categorized into several super clades. (b) Thirty-three putative effector genes are aggregated into 11 clusters with two to six effector genes. Shaded arrows represent putative effector genes while white arrows are for other genes. (c) Microsynteny analyses betweenU. virensandM. anisopliaegenomes revealed that most of effector gene clusters lie in the highly diverse genomic regions flanked by conserved sequences. Shaded arrows are putative effector; brick red represents homologous proteins with >80% amino-acid identity; yellow, 60~80% amino-acid identity; green, <60% identity; and white, no homologous proteins revealed by genome comparisons using SyMAP v4.0. Three effector gene clusters are shown here, others are shown inSupplementary Fig. 9. (d–h) Physical locations of predicted secreted protein genes, all protein-coding genes and PHI-base genes in relation to regions of repetitive sequences and GC content distribution in the assembled genome ofU. virens(using scaffold #1 as an example). (d) Locations of genes encoding predicted secreted proteins (purple) including putative effectors (indicated by red arrows) in the assembled genome. (e) The distribution of transposable elements (blue) in theU. virensgenome. (f) Single-copy DNA regions (red) of theU. virensgenome. (g) Locations of the PHI-base gene homologues (green) involved in pathogen–host interactions. (h) Graphs of GC (red) and AT (blue) contents. Areas of low GC correspond well to the regions of repetitive DNA. The maps fromd–gwere drawn with OmniMapFree. Repetitive elements affected by RIP and RNA silencing A total of 160 repetitive families including 10 families of DNA transposons, 45 long terminal repeat (LTR) and 6 non-LTR retrotransposons were identified in U. virens ( Supplementary Table 5 , Supplementary Note 2 ). These repeat families account for ~25% of the genome ( Fig. 2a ). The majority of repetitive sequences (~72%) are transposable elements (TEs), and the remaining are simple sequence repeats. LTR retrotransposons represent about 83% of TEs. DNA transposons include Helitrons that account for ~50% of DNA transposons, one terminal inverted repeat family, and some undefined families ( Fig. 2a ). Figure 2: Repetitive sequences have been affected by repeat-induced point mutations in U. virens . ( a ) The proportion (%) of different types of repetitive sequences in the U. virens UV-8b genome. ( b ) Estimation of RIP for five sequenced ascomycete genomes. Average RIP indices in U. virens, F. graminearum, M. oryzae, N. crassa and M. anisopliae and the ratio of each type of di-nucleotide (ratio of frequency in repetitive elements to that in non-TEs) in different fungal genomes are shown. Full size image RIP (repeat-induced point mutation) is a genome defence mechanism in fungi that might prevent gene creation through genomic duplication [26] . A high ratio of TpA/ApT (1.48) and a low value for (CpA+TpG)/(ApC+GpT) (<1.0) were observed, implying strong RIP in U. virens ( Supplementary Note 2 ). The high average ratio of di-nucleotide preference also provides genome-level evidence for the efficiency of RIP. U. virens has a di-nucleotide ratio index similar to N. crassa and higher than other sequenced ascomycetes ( Fig. 2b ), which indicates that RIP, similar to that found with N. crassa genome, is a significant characteristic of U. virens genome. Furthermore, alignment of homologous TEs revealed numerous point mutations representing C-to-T (G-to-A) transitions in the TE sequences, implying that RIP can also control TE activity in U. virens ( Supplementary Fig. 2 ). The active RIP defence mechanism in U. virens is also supported by the presence of a DNA methyltransferase RID (for RIP defective) homologue, a key protein in the RIP machinery in N. crassa . RNA silencing is well recognized as a principal regulatory mechanism in eukaryotes to control gene expression [27] . 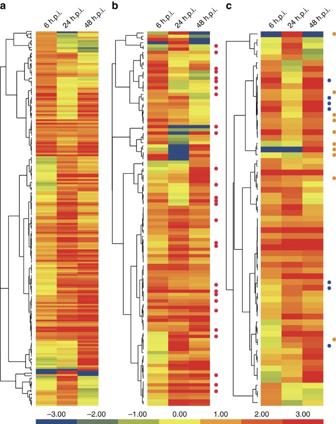Figure 6: The expression pattern of upregulated PHI-base genes and genes for secreted proteins and secondary metabolism duringU. virensinfection. (a) A total of 213 genes involved in pathogen–host interactions were upregulated at 6 h, 24 h and 48 h post inoculation (h.p.i.). (b) A total of 116 genes encoding predicted secreted proteins including 28 putative effectors were upregulated at 6 h.p.i., 24 h.p.i. and 48 h.p.i. Red dots indicate putative effector proteins. (c) A total of 65 genes involved in secondary metabolic processes were transcriptionally induced at 6 h.p.i., 24 h.p.i. and 48 h.p.i. Blue dots indicate predicted PKS/PKS-like proteins; yellow dots indicate predicted NRPS/NRPS-like proteins. These genes are significantly enriched in the upregulated genes during early stages ofU. virensinfection. Hierarchical clustering analysis was performed for these transcripts at 6 h.p.i., 24 h.p.i. and 48 h.p.i. Each column represents the fold change in transcript levelsin plantaat the indicated times, relative to the levelsin vitro. The vertical dimension represents genes that exhibited changes in transcript level (cutoff: |log2[fold change]|⩾1 and false discovery rate≤0.001). The colour scale indicates transcript abundance relative to the mycelium before inoculation: red, increase in relative transcript abundance; blue, decrease in relative transcript abundance. The key genes necessary for RNA silencing pathways are highly conserved in U. virens including three Argonaute-like proteins required for forming RNA-induced silencing complex, three RNA-dependent RNA polymerases, three ReqQ helicases and two Dicer genes ( Supplementary Table 6 ). 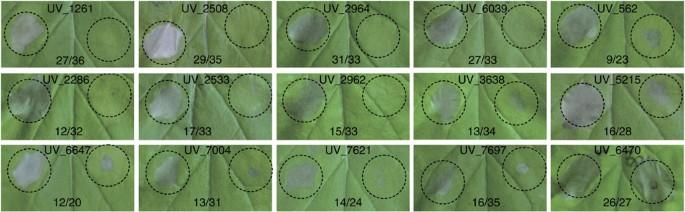Figure 7: PutativeU. virenseffectors suppressedB. glumae-induced HR inN. benthamiana. Representative cell death symptoms were photographed at 2–3 days afterB. glumaeinoculation. The left half leaf sections were injected withB. glumaewith the pEDV empty vector and the right half sections were injected withB. glumaewith effector gene constructs. Numbers, for instance 27/36, indicate that the 27 right leaf sections out of 36 inoculated leaves showed no or significantly less severe symptoms as compared with left sections. These genes are speculated to function in two fungus-specific RNA-silencing pathways: meiotic silencing of unpaired DNA and quelling ( Supplementary Table 7 ). Comparative genomics and evolution Four additional strains collected from different geological regions in China ( Supplementary Table 8 ) were subjected to low-depth sequencing for comparative genomics. Microsynteny analyses at the mating-type loci among the five strains indicated that each U. virens genotype has only a single mating-type locus and that U. virens is heterothallic ( Supplementary Fig. 3 , Supplementary Note 3 ). Comparison with the reference genome of UV-8b revealed low rate of single nucleotide polymorphisms among all these strains. The relatively low nucleotide diversity between genotypes indicates a low level of intraspecific sequence variation, suggesting a recent expansion of the U. virens population ( Supplementary Table 9 , Supplementary Note 4 ). The ratio of nonsynonymous to synonymous substitutions (Ka/Ks) was calculated to assess selection pressures on U. virens evolution from the host interaction. In the UV-8b strain versus the four other strains, 2,957 and 1,451 genes were found to have nonsynonymous and synonymous substitutions, respectively; 286 genes have both nonsynonymous and synonymous substitutions, of which 277 genes have a Ka/Ks<1 and only nine genes have a Ka/Ks>1 ( P <0.05) ( Supplementary Data 1 ). Among these are five effector-like genes and three with putative functions in DNA repair and cell cycle regulation ( Supplementary Note 4 ). The phylogenetic position of U. virens was evaluated among other eleven selected fungal species (10 ascomycota and one basidiomycota outgroup) using a set of highly conserved single-copy genes suggested for the Fungal Tree of Life [28] ( Supplementary Table 10 , Supplementary Note 5 ). The analysis revealed that U. virens is more closely related to two entomopathogenic Metarhizium spp. (Hypocreales, Clavicipitaceae) than to other species including the plant pathogen Claviceps purpurea (Hypocreales, Clavicipitaceae) and the insect pathogenic fungus Cordyceps militaris (Hypocreales, Clavicipitaceae) ( Fig. 3 ). Furthermore, U. virens shares more homologous proteins with >60% identity and more identical amino-acid positions with Metarhizium spp. than with the other tested fungi. Proteome comparisons also revealed a 10.7–11.1% greater amino-acid similarity of U. virens to Metarhizium spp. than to C. purpurea ( Supplementary Table 11 ). Comparative genomic analyses revealed that U. virens shares more reciprocal best hit orthologous genes with M. acridum (5,702) and M. anisopliae (5,644) than with the other species, although by this metric Fusarium graminearum shared a surprisingly high 5,639 orthologous genes with U. virens ( Supplementary Table 11 ). Synteny analysis also showed that U. virens and M. anisopliae genome structures have many large areas of synteny ( Supplementary Fig. 4 ). Figure 3: Phylogenetic analyses for evolutionary relationships among different fungi. The fungi are U. virens, C. purpurea, M. anisopliae, M. acridum, C. militaris, M. oryzae, F. graminearum, N. crassa, A. fumigatus, S. cerevisiae, S. sclerotiorum and U. maydis . A maximum likelihood phylogenetic tree constructed based on derived protein sequences of 21 single-copy genes common to these 12 fungal genomes that were identified from a set of 74 single-copy orthologous genes across the Kingdom Fungi showing evolutionary relationships among these fungi. Full size image Comparisons among U. virens , Magnaporthe oryzae , F. graminearum and M. anisopliae genomes were performed to identify genes that are absent from the U. virens genome since it has a smaller gene inventory. A total of 703 orthogroups were identified, 486 of which have gene ontology (GO) annotations. Interestingly, the majority of missing orthogroups belong to the GO terms in molecular functions (4) and in biological processes (11; see Supplementary Table 12 ). A significant reduction was observed in proteins for oxidoreductase activity, proteins related to toxin and secondary metabolism, energy metabolism and catabolism and responses to toxin and chemical stimuli ( Supplementary Table 12 ). Weakened polysaccharide degradation machinery For successful infection, phytopathogenic fungi often have to break down plant cell walls by carbohydrate-active enzymes including glycoside hydrolases, glycosyl transferases, polysaccharide lyases (PL) and cutinases. Interspecific comparisons showed that U. virens encodes significantly fewer carbohydrate-active enzymes than plant hemi-biotrophic fungi, such as M. oryzae and F. graminearum . Particularly, the proteins in such families as GH6, GH7, GH39 and GH51 that are involved in degrading cellulose, hemi-cellulose and pectin of plant cell walls are significantly reduced in comparison with M. oryzae and F. graminearum ( P <0.01; Supplementary Tables 13, 14 , Supplementary Note 6 ). This characteristic is similar to the obligate biotrophic powdery mildew and entomopathogenic fungi that have no canonical plant cell wall-degrading enzymes [29] . Corresponding to these findings, putative carbohydrate-binding proteins are significantly reduced in U. virens ( Supplementary Table 15 ). Distinctively, the fungus seems to lack PLs including pectin lyases and pectate lyases ( Table 2 ). Consistently, other enzymes involved in pectin degradation are less frequent or absent, such as the d-4,5 unsaturated α-glucuronyl hydrolase GH105 family that can sequentially degrade the products generated by PLs ( Supplementary Table 13 ) [30] . Furthermore, U. virens contains fewer putative cutinases needed for plant cuticle degradation ( Table 2 ). Collectively, these analyses suggest that polysaccharide degradation machinery is compromised in U. virens and degrading plant cell wall is probably not essential in establishing infection. Table 2 Selected protein families involved in fungal pathogenesis in U. virens and other ascomycetes. Full size table To verify the results from bioinformatic analyses, the pectinolytic activities of U. virens were evaluated in comparison with M. oryzae , F. graminearum and Colletotrichum fragariae ( Supplementary Note 6 ). As predicted by genomic data that U. virens has very limited abiltiy to secrete pectin-degrading enzymes, no translucent area indicating of pectin degradation was observed for U. virens, while a clear transparent halo was formed in the C. fragariae -cultured plates ( Supplementary Fig. 5a ). In addition, U. virens grew well in the medium using glucose or sucrose as sole carbon, while it did not grow at all on pectin and grew poorly on xylan and cellulose. In contrast, C. fragariae and Rhizoctonia solani grew rapidly on pectin plates ( Supplementary Fig. 5b ). Pectinolytic activity assays and carbon growth profiles of U. virens supported the bioinformatic prediction. Reduced G-protein-coupled receptors and transporters In phytopathogenic fungi, G-protein-coupled receptors (GPCRs) and G-proteins are important components of signalling pathways for response to environmental stimuli [31] . U. virens , similar to the non-pathogenic saprophyte N. crassa , encodes fewer GPCRs than the hemi-biotrophic pathogens M. oryzae and F. graminearum ( Supplementary Table 16 , Supplementary Note 7 ). In particular, U. virens contains many fewer Pth11 homologues that are required for appressorium differentiation in response to host surface stimuli and pathogenesis [32] . No homologues of Saccharomyces cerevisiae GPR1, the sucrose/glucose sensing receptor, were predicted in U. virens [33] . Significant loss of GPCRs suggests that the biotrophic U. virens , adapted to a narrow niche for host infection, might use specialized receptors for extracellular signals compared with the hemi-biotrophic M. oryzae and F. graminearum . In addition, U. virens has more β-subunits of G-proteins ( Supplementary Table 17 ). U. virens also encodes significantly fewer transporters, including members in the amino-acid-polyamine-organocation, ATP-binding cassette and major facilitator superfamilies (MFS). In contrast, the proteins in the oxidoreduction-driven transporter subclass are expanded ( Supplementary Table 18 , Supplementary Note 7 ). Many MFS transporters are involved in the transport of a wide range of nutrient substrates, such as sucrose, galactoside, amino acid and peptides [34] . Reduced MFS transporters and lack of the nutrient sensor GPR1 suggest that U. virens might have a narrow specificity to utilize nutrients from host plants. Secondary metabolism genes U. virens genome encodes 17 non-ribosomal peptide synthetases (NRPS), 14 polyketide synthases (PKS), 6 geranylgeranyl diphosphate synthases, 6 terpene synthases, and 6 terpenoid cyclases. These enzymes are responsible for fundamental steps in the biosynthesis of secondary metabolites, such as mycotoxins, alkaloids and pigments ( Supplementary Table 19 , Supplementary Note 8 ). However, U. virens lacks dimethylallyl tryptophan synthases, which catalyse the first committed step of ergot alkaloid biosynthesis [35] . In M. robertsii , the NRPS protein DtxS1 with six adenylation domains is responsible for the biosynthesis of the cyclic hexadepsipeptide destruxins, which are structurally similar to ustiloxins [36] . Of the predicted NRPS/NRPS-like proteins, UV_1490 and other five have adenylation domain(s) that recognize the cognate amino-acid substrate and activate it as its aminoacyl adenylate for peptide synthesis ( Supplementary Table 20 ). These NRPS/NRPS-like genes are within clusters with genes encoding acyltransferases, dehydrogenases (DHGs), oxidoreductases and/or cytochrome P450s (CYPs) involved in the modification of secondary metabolites ( Fig. 4a and Supplementary Fig. 6 ), suggesting that one or more of them may be responsible for the synthesis of ustiloxins. The core structure of ustilaginoidins is formed by dimerization of nor-rubrofusarin that is an intermediate during aurofusarin biosynthesis in F. graminearum [12] , [37] . Through comparisons with the identified aurofusarin biosynthesis gene cluster [37] , the PKS gene cluster that may be responsible for the biosynthesis of ustilaginoidins was also found in U. virens ( Fig. 4b , Supplementary Table 21 and Supplementary Note 8 ). Figure 4: Putative NRPS and PKS gene clusters for ustiloxin and ustilaginoidin biosynthetic pathways. ( a ) The putative NRPS gene (central long red arrow) cluster for ustiloxin biosynthesis. UV_1490 containing three adenylation domains may be responsible for the biosynthesis of the core structure of ustiloxins. The NRPS gene is clustered around genes encoding dehydrogenase, oxidase, monooxygenase and transcription factor that may be involved in the modification of secondary metabolites. ( b ) Comparison between the putative PKS gene cluster for ustilaginoidin biosynthesis in U. virens (upper) and the aurofusarin biosynthesis gene cluster in F. graminearum (bottom). The UV_2086 ( PKS ), UV_2087 , aurT and gip1 genes (green) in U. virens were identified by BLASTing against the aurofusarin biosynthesis genes while other genes (purple) were predicted via Pfam domain search. The aurF and aurL2 genes (grey) in the aurofusarin biosynthesis gene cluster in F. graminearum are absent in U. virens genome. Full size image Molybdoprotein biosynthesis and nutrient uptake pathways, such as thiamine biosynthesis play vital roles in lifestyle of pathogenic fungi [38] . The genes involved in these biosynthesis pathways were compared among U. virens and some obligate biotrophs, hemibiotrophs and necrotrophs to better understand evolution to biotrophy ( Supplementary Note 8 ). Components of these pathways were partially found in the genomes of the biotrophs U. virens , U. maydis , Blumeria graminis and Puccinia striiformis ( Supplementary Table 22 ), suggesting that loss of thiamine and molybdoprotein biosynthetic pathways is likely the result, but not the reason for biotrophy in fungi [38] . Important gene families involved in pathogenicity To investigate pathogenicity genes in U. virens , virulence-associated mitogen-activated protein kinase (MAPK) cascades were first surveyed. Multiple analyses indicated that U. virens might contain five MAPK pathways similar to S. cerevisiae and that MAPK signalling pathways were highly conserved in phytopathogenic fungi ( Supplementary Figs 7, 8 , Supplementary Table 23 , Supplementary Note 9 ). Furthermore, genome-wide BLAST analyses against PHI-base [20] , which includes experimentally verified genes involved in pathogen–host interactions revealed that 1,103 protein-coding genes in U. virens were putatively involved in virulence and pathogenicity, which account for 13.1% of the total predicted genes ( Table 2 , Supplementary Table 24 , Supplementary Note 9 ). Proteins identified in PHI-base as involved in secondary metabolism, degradation enzymes for large molecules that might be involved in breaking host physical barriers, MFS and ATP-binding cassette transporters, DHGs and CYPs, and some transcription factors in U. virens were less abundant than those in M. oryzae and F. graminearum ( Supplementary Tables 24,25 ). In contrast, many protein families in PHI-base that are considered essential for basic cellular processes, such as DNA/RNA helicases, DNA topoisomerase and DNA-directed DNA polymerases, are conserved in U. virens ( Supplementary Table 24 ). GLEYA adhesin, CheY-like proteins and proteins secreted in xylem are even expanded in PHI-base of U. virens as compared with F. graminearum or M. oryzae ( Table 2 , Supplementary Table 24 , Supplementary Note 9 ). U. virens secretome and effector prediction The proteins secreted by pathogenic fungi, particularly effectors, are among essential components for successful infection, especially for the biotrophic fungi that have intimate host–fungal interactions [39] . U. virens genome encodes 628 (527 without transmembrane domains) potentially secreted proteins, including 193 small (<400 amino acids), cysteine-rich ( ⩾ 4 cysteine residues) proteins that are putative effectors ( Fig. 5a , Supplementary Note 10 ). Figure 5: Genes and gene clusters encoding putative effectors and their locations in relation to repetitive sequences in the U. virens genome. ( a ) A phylogenetic tree of 193 putative effectors indicates that most effectors are categorized into several super clades. ( b ) Thirty-three putative effector genes are aggregated into 11 clusters with two to six effector genes. Shaded arrows represent putative effector genes while white arrows are for other genes. ( c ) Microsynteny analyses between U. virens and M. anisopliae genomes revealed that most of effector gene clusters lie in the highly diverse genomic regions flanked by conserved sequences. Shaded arrows are putative effector; brick red represents homologous proteins with >80% amino-acid identity; yellow, 60~80% amino-acid identity; green, <60% identity; and white, no homologous proteins revealed by genome comparisons using SyMAP v4.0. Three effector gene clusters are shown here, others are shown in Supplementary Fig. 9 . ( d – h ) Physical locations of predicted secreted protein genes, all protein-coding genes and PHI-base genes in relation to regions of repetitive sequences and GC content distribution in the assembled genome of U. virens (using scaffold #1 as an example). ( d ) Locations of genes encoding predicted secreted proteins (purple) including putative effectors (indicated by red arrows) in the assembled genome. ( e ) The distribution of transposable elements (blue) in the U. virens genome. ( f ) Single-copy DNA regions (red) of the U. virens genome. ( g ) Locations of the PHI-base gene homologues (green) involved in pathogen–host interactions. ( h ) Graphs of GC (red) and AT (blue) contents. Areas of low GC correspond well to the regions of repetitive DNA. The maps from d – g were drawn with OmniMapFree. Full size image Among them, 34 predicted effector genes are organized into clusters/families containing two to six related genes, suggesting that local duplications might be involved in expansion of effectors in U. virens ( Fig. 5a,b ). In the maize pathogen U. maydis , some effector gene clusters play decisive roles through the course of infection [40] . Among these recently expanded U. virens effectors, we observed surprisingly low Ka/Ks ratios and low SNP frequency among five sequenced strains, suggesting a low intraspecific genetic diversity among the pathogen population, even for the fast evolving effectors ( Supplementary Table 9 and Supplementary Data 1 ). However, when comparing with the close evolutionarily related fungal species Metarhizium spp. ( Fig. 3 ), we observed accelerated interspecific diversification. For instance, pairwise comparisons showed that over 63% of non-secreted proteins in U. virens shared >60% amino-acid identity with those in either M. anisopliae or M. acridum , respectively. In contrast, predicted secreted proteins share significantly lower amino-acid identity between these species. More evidently, only 43 and 40 putative effector proteins (22.3% and 20.7%) in U. virens share high amino-acid identity (>60%) with the protein inventory in M. anisopliae and M. acridum , respectively ( Supplementary Table 26 ). Microsynteny analyses between U. virens and M. anisopliae were performed for 11 putative effector gene clusters. Seven clusters containing 24 putative effectors were found in highly diverse genomic islands flanked by conserved regions ( Fig. 5c and Supplementary Fig. 9 ). These results imply that secreted proteins, especially effector proteins, have evolved more rapidly than other proteins in U. virens and that these proteins may play important roles in host adaptation. Repetitive elements often play important roles in genome evolution, including birth/death and diversification of functional genes such as effector genes, secondary metabolite biosynthesis genes [35] , [41] . However, no direct correlation between candidate effectors and TE-rich regions (low GC content) was evident in the U. virens genome ( Fig. 5 ). This result suggests that TE-driven evolution might have less of an effect on the synergistic interactions of U. virens and rice than on some other host–pathogen interactions, such as M. oryzae and rice [35] , [41] . Transcriptome profiles during early infection To understand pathogenicity and in planta transcriptional reprogramming, gene-expression profiles of U. virens were studied during early infection. As compared with axenic cultures, 830, 497 and 484 genes were upregulated while 452, 224 and 266 genes were downregulated at 6, 24 and 48 h post inoculation (h.p.i. ), respectively ( Supplementary Fig. 10 ). A total of 1,319 upregulated genes and 687 downregulated genes were identified during early stages of U. virens infection ( Supplementary Fig. 11 and Supplementary Data 2 ). GO enrichment analyses revealed that the majority of the very early specifically induced genes (at 6 h.p.i.) were enriched in the cellular component terms while the upregulated genes at slightly later stages (at 24 and 48 h.p.i.) were mainly enriched in the biological process and biological function terms ( Supplementary Table 27 ). Four categories of important virulence-associated genes were identified to be highly induced during infection. First, 213 PHI-base genes are upregulated in infected rice panicles ( Fig. 6a ). Particularly, 21 PHI-base genes are among the top 100 most highly induced genes ( Supplementary Table 28 ), indicating an important role of these PHI-base genes in the interaction with host rice. Second, 15 secreted protein genes including 5 putative effector genes are significantly enriched in the top 100 most highly induced genes ( P <0.01; Supplementary Table 28 and Fig. 6b ). Among the induced secreted proteins, some putative effectors with conserved functional domains such as fungal-specific extracellular EGF-like (CFEM), WSC, necrosis-inducing protein, ribonuclease, LysM, glycoside hydrolase or peptidase domains might play significant roles in fungal pathogenesis. Third, the secondary metabolism genes including 10 NRPS/NRPS-like, 7 PKS/PKS-like genes and many methyltransferase, acetyltransferase, carboxylesterase and CYP genes are significantly enriched in the transcriptome ( P <0.01; Fig. 6c , Supplementary Table 27 ), implying essential roles of mycotoxins during early infection of U. virens . Fourth, a set of plant specifically expressed genes were identified, among which putative effector genes are enriched ( Supplementary Table 29 ). Interestingly, most of the plant-specific expressed genes have no known function(s) with characteristics of effectors. Figure 6: The expression pattern of upregulated PHI-base genes and genes for secreted proteins and secondary metabolism during U. virens infection. ( a ) A total of 213 genes involved in pathogen–host interactions were upregulated at 6 h, 24 h and 48 h post inoculation (h.p.i.). ( b ) A total of 116 genes encoding predicted secreted proteins including 28 putative effectors were upregulated at 6 h.p.i., 24 h.p.i. and 48 h.p.i. Red dots indicate putative effector proteins. ( c ) A total of 65 genes involved in secondary metabolic processes were transcriptionally induced at 6 h.p.i., 24 h.p.i. and 48 h.p.i. Blue dots indicate predicted PKS/PKS-like proteins; yellow dots indicate predicted NRPS/NRPS-like proteins. These genes are significantly enriched in the upregulated genes during early stages of U. virens infection. Hierarchical clustering analysis was performed for these transcripts at 6 h.p.i., 24 h.p.i. and 48 h.p.i. Each column represents the fold change in transcript levels in planta at the indicated times, relative to the levels in vitro . The vertical dimension represents genes that exhibited changes in transcript level (cutoff: |log 2 [fold change]| ⩾ 1 and false discovery rate≤0.001). The colour scale indicates transcript abundance relative to the mycelium before inoculation: red, increase in relative transcript abundance; blue, decrease in relative transcript abundance. Full size image Functional studies on putative effectors Plant pathogenic fungi often overcome host immunity through the action of effector proteins [42] . To experimentally identify novel U. virens effectors, a pEDV-based screen was performed for 30 randomly selected putative effectors in which a type III secretion system of the emerging rice pathogen Burkholderia glumae was used to translocate these putative secreted proteins into plant cells to identify effectors that suppress hypersensitive responses (HR) in Nicotiana benthamiana [43] . The screen showed that 4 out of the 30 putative effectors such as UV_2964 had very strong HR suppressive ability, 4 including UV_5215 had a strong suppressive effect, 10 effectors had a weak effect, and others, for example, UV_6470 had little or no effect on inhibiting HR in N. benthamiana ( Fig. 7 , Supplementary Table 30 ). Among them, UV_6647 and UV_2799 are upregulated during early infection, UV_5215 is a plant-specific expression gene, and UV_2962 and UV_2964 are within the same gene cluster ( Fig. 5b ). Interestingly, UV_2286 encodes a peptide highly similar to Hirsutellin A, an insecticidal ribotoxin produced by Hirsutella thompsonii [44] . UV_6647 encodes a homologue to phosphohistidine phosphatase SixA from Escherichia coli that modulates the ArcB phosphorelay signal transduction [45] . Figure 7: Putative U. virens effectors suppressed B. glumae -induced HR in N. benthamiana . Representative cell death symptoms were photographed at 2–3 days after B. glumae inoculation. The left half leaf sections were injected with B. glumae with the pEDV empty vector and the right half sections were injected with B. glumae with effector gene constructs. Numbers, for instance 27/36, indicate that the 27 right leaf sections out of 36 inoculated leaves showed no or significantly less severe symptoms as compared with left sections. Full size image U. virens has been recognized as the fastest spreading and economically important pathogen on rice [5] , [17] . In this study, we sequenced, assembled and analysed the draft genome of this important pathogen. U. viren s has a genome size of 40.4 Mb, which is in the midrange of 15 plant-associated Clavicipitaceae fungal genomes from 28.9–58.7 Mb, with large variations in repeat sequences [35] . The genome contains ~25% repeat sequences, most of which are TEs. Multiple analyses indicate that U. virens , similar to N. crassa , uses RIP, a fungus-specific genome defence mechanism [46] to control TE activity ( Fig. 2 , Supplementary Fig. 2 ). U. virens also possesses orthologues of all the N. crassa genes postulated to be involved in RNA silencing ( Supplementary Table 6 ). This suggested that both RNA silencing and RIP are involved in defence against adverse effects of proliferating repetitive sequences in U. virens . As the only sequenced fungal species in the tribe Ustilaginoideae, the U. virens genome provides useful information on host adaptation and evolutionary relationships in the Hypocreales. Comparison of U. virens with several Hypocreales and some other important plant pathogens showed that U. virens is evolutionarily close to the entomopathogenic Metarhizium spp., as assessed by multiple criteria, suggesting a host shift across the plant and animal kingdoms. Recently, Metarhizium spp. was found to be phylogenetically closer to plant pathogens than to the animal pathogens A. fumigatus and C. albicans [34] . Spatafora et al . [47] showed phylogenetic relationships among members of tribe Ustilaginoideae and hypothesized an animal pathogen origin for the ergot and grass endophytes. According to the host habitat hypothesis [18] , U. virens might have evolved from an entomopathogenic fungus because of their co-occurrence in the same environment. Our comparative genomics analyses found that U. viren s contains many fewer genes than hemi-biotrophic fungal pathogens including F. graminearum and M. oryzae or the necrotrophic S. sclerotiorum [48] . In particular, U. virens is dramatically reduced in at least three categories of functional proteins. First, U. virens has a smaller inventory of carbohydrate-active enzymes with almost no ability to degrade pectin and a very low capability to break down cellulose and xylan ( Table 2 , Supplementary Fig. 5 ). These results indicate that U. virens with its biotrophic lifestyle may minimize the release of cell wall fragments by carbohydrate-active enzymes, whose products are often recognized as endogenous signals to induce plant immunity [38] , [40] . The smaller polysaccharide degradation machinery and other genomic features also reflect the infection pattern of U. virens that infects plants through stamen filaments where cell wall materials such as cellulose and pectin are deficient [17] . Second, U. virens contains many fewer MFS transporters that have been reported to be mainly associated with nutrient uptake and antifungal drug resistance [49] . Furthermore, the genome was not found to encode GPR1 nutrient sensors and has many fewer proteins involved in energy metabolism ( Supplementary Tables 12,16 ). During floral infection, the fungus does not form haustoria [17] , the structure involved in nutrient uptake for many biotrophs. Taken together, these characters indicated that U. virens may have a limited ability to acquire nutrients from plant tissues and organs. Abundant and easily obtained nutrients in the male flower parts including pollens may contribute to primary colonization of U. virens in the rice florets. Third, DHGs, CYPs and other enzymes involved in secondary metabolism are significantly fewer ( Table 2 , Supplementary Table 24 ). CYPs on both flanks of NRPSs and PKSs are also much less abundant than those in M. anisopliae . DHGs and CYPs in phytopathogenic fungi contribute to detoxification of phytoalexin repertoires of host plants [50] . The smaller inventory of CYPs and DHGs indicates that U. virens may have a lower capacity for adaptation to different plants, which may explain the relatively narrow host range of U. virens . Despite a reduced secondary metabolism gene inventory, many genes involved in secondary metabolism including more than half of NRPS and PKS genes were greatly induced in planta during infection ( Fig. 6c and Supplementary Data 2 ). This is consistent with the observation that ustiloxin is easily extracted from spore balls, but not from axenic cultures. Therefore, we hypothesize that secondary metabolites, particularly mycotoxins might act as virulence factors during infection. The predicted ustiloxin and ustilaginoidin biosynthesis gene clusters provide the foundation to test such hypotheses experimentally. In planta expression profiles also indicated that a set of secreted protein and PHI-base genes are important for pathogenicity of U. virens . In particular, many effector candidates were highly upregulated during infection ( Fig. 6b ). They include secreted in xylem proteins, peptidases, ribonucleases, glycosyl hydrolases and other proteins with the typical effector domains, such as NPP1, CFEM and WSC, which have been found to play significant roles in fungal pathogenesis ( Supplementary Data 2 ). We experimentally demonstrated that more than half of randomly selected putative effectors could suppress B. glumae -triggered HR in N. benthamiana to different degrees ( Fig. 7 ). The results indicated that these effectors may play essential roles in shaping the interaction of U. virens with its host. Predicted secreted proteins, particularly putative effector proteins, are highly diverse between U. virens and M. anisopliae despite their close evolutionary relationship ( Supplementary Table 26 ). Consistently, the effector gene clusters in U. virens are predominantly located in highly diverse genome regions when aligned with the M. anisopliae genome ( Fig. 5c and Supplementary Fig. 9 ). These analyses suggest that adaptation to distinct hosts across kingdoms might result in divergent effector repertoires. However, within species these putative U. virens effector genes are highly conserved. We thus hypothesize that a recent founder effect has occurred in U. virens , and perhaps a virulent U. virens strain, which emerged and established intimate interactions with rice rather recently, spread rapidly thereafter. Over a short co-evolutionary history, effector-triggered host immunity has not evolved to suppress pathogen invasion and therefore effectors have been subjected to little selection pressure. No gene-for-gene resistance has been reported for the rice– U. virens pathosystem yet [5] , which supports the hypothesis. In summary, we reveal the close evolutionary relationship between U. virens and Metarhizium spp., implying that the Clavicipitaceae fungi exhibit host shifting across plant and animal kingdoms. Besides, we hypothesize that low intraspecific genetic diversity in U. virens is perhaps attributable to a recent founder effect. Significant fewer gene inventories involved in cell wall degrading, nutrient uptaking and secondary metabolism reflect a biotrophic lifestyle and flower filament infection style of U. virens . Functional studies together with transcriptome and microsynteny analyses indicate that putative effectors play important roles in virulence, pathogenicity and host adaptation. Together, our comparative and functional genomics analyses offer new insights into molecular mechanisms of evolution, biotrophy and pathogenesis of U. virens , and lay the groundwork for future discoveries with this increasingly important plant pathogen. DNA isolation and rice inoculation Ustilaginoidea virens strains UV-8b, FJ1-1a, HB3-1a, LN10-16-1 and LN2010-1-1 were collected from different rice cultivars at different provinces in China, and used for sequencing ( Supplementary Table 8 ). Total DNA was isolated from the mycelium of U. virens using a CTAB (cetyl trimethyl ammonium bromide) method [51] . Nuclear DNA was purified through a CsCl density-gradient centrifugation to remove mitochondrial DNA using standard procedures [52] . Rice plants of the cultivar LYP9 that is highly susceptible to RFS were inoculated with conidial suspensions as described with some modifications [53] . Briefly, the U. virens monoconidial cultures were grown in potato sucrose broth in an incubator shaker at 150 r.p.m. at 28 °C for 5 days. About 1 ml of conidial suspension (2 × 10 5 conidia ml −1 ) was injected into the leaf sheaths of field grown rice plants at the booting stage 5–7 days before heading. This was done in the late afternoon with a suitable temperature for better infection. The panicles were harvested at 6 h, 24 h and 48 h post inoculation (h.p.i. ), frozen immediately in liquid nitrogen, and then kept at −70 °C for RNA isolation. Genome sequencing and assembly The UV-8b genome was sequenced with the Roche 454 sequencing platform at Sun Yat-sen University, Guangzhou, China. DNA libraries with 500 bp and 5 kb inserts were subsequently constructed for UV-8b and libraries with 500 bp inserts were constructed for the four other U. virens strains. These DNA libraries were 100 bp paired-end sequenced using the Illumina HiSeq2000 at the Beijing Genomics Institute (BGI) in Shenzhen, China. Genome assembly for 454 data was done with Newbler (version 2.5, Roche) using the default parameters. Data from the Illumina libraries were first trimmed by removing bases with quality score below 20 at both ends and discarding trimmed reads with lengths less than 70 bp. The Newbler contigs were used as single-end data and fed into the ABySS [21] version 1.2.7 assembly pipeline along with the paired-end Illumina data for strain UV-8b. The contigs generated by ABySS were processed with SSPACE scaffolder to construct scaffolds [22] . All of the available paired-end reads were mapped to previously generated contigs to connect adjacent contigs through paired-end data from the 500 bp and 5 k libraries. Larger scaffolds were then made using GapCloser [54] to complete the whole-genome sequence of U. virens . The genome size of U. virens was estimated from the UV-8b sequencing data using JELLYFISH (Version 2.0) [23] . Gene annotation Protein-coding genes in U. virens were predicted independently with three ab initio predictors SNAP, GeneMark+ES and AUGUSTUS [55] , [56] , [57] . The accuracy of ab initio annotation was then improved using RNA-seq data from U. virens and from the proteomes of nine sequenced fungi. The RNA-seq data were aligned to the U. virens UV-8b genome through TopHat [58] , and potential transcripts in U. virens genome were predicted using Cufflinks [59] . The nine sequenced fungal proteomes were aligned to the U. virens genome by TBLASTN [60] . Proteins with sequence identity more than 70% were noted and used as templates to predict the exons of U. virens genes with Genewise [61] . Subsequently, the outputs from these three methods were transformed to GFF file with local PERL scripts. The resultant GFF files from each of the prediction programs were used as input into the EVM program to integrate the three sources of gene predictions [62] . SNP identification and Ka/Ks calculation Genome sequencing reads of the four U. virens strains were mapped onto the U. virens UV-8b reference genome using SOAP2 ( http://soap.genomics.org.cn/soapaligner.html ) with default settings. SNPs were identified through the comparison with the reference by SOAPsnp ( http://soap.genomics.org.cn/soapsnp.html ). For Ka/Ks calculation, sequence reads were mapped to the coding sequences of the 8,426 predicted genes of the UV-8b reference strain and thus obtaining consensus CDS sequences that were aligned with ClustalW2 (ref. 63 ). The fasta files with aligned sequences were converted into AXT files by parseFastaIntoAXT.pl ( http://code.google.com/p/kaks-calculator/ ) and ratios of Ka and Ks were calculated using the Modified YN method [64] . The Fisher’s exact test was used to obtain P -values in this calculation. RNA-Seq and transcriptome analyses Total RNA was isolated from in vitro cultures and from inoculated rice panicles using RNApure RNA isolation kit according to the manufacturer’s instructions (Aidlab Biotechnologies, Beijing). RNA integrity was confirmed using the 2100 Bioanalyzer (Agilent Technologies) with a minimum RNA integrity number (RIN) value of 7. Total RNA from three biological replicates at each time point (6 h.p.i., 24 h.p.i. and 48 h.p.i.) were combined and used for library construction. All procedures, including mRNA purification, cDNA preparation, end repair of cDNA, adaptor ligation and cDNA amplification were carried out following BGI standard methods for preparing Illumina RNA-seq libraries. Each library had an insert size of ~200 bp. The reads of 49 bp (for in planta expression profiling) or 100 bp (for transcriptome analysis of in vitro cultures) sequences were generated via Illumina HiSeq2000 at BGI. Raw image data were transformed into sequence data by base calling. All sequences were filtered to remove adaptor sequences and low-quality sequences (where the percentage of the low-quality bases with quality value ≤5 was greater than 50% in a read). The quality-trimmed reads were mapped to U. virens genome using SOAP aligner/SOAP2, allowing up to two base mismatches per read. The RPKM (reads per kb per million reads) was calculated to reflect the expression level of U. virens transcripts in planta [65] . To compare the differences in gene expression, differentially expressed genes were identified with the criterion of the absolute log 2 ratio value ⩾ 1 and false discovery rate ≤0.001 (ref. 66 ). Secreted proteins and potential effector analysis Potential secreted proteins in U. virens were predicted using SignalP 4.0 (ref. 67 ). Putative effectors in the U. virens secretomes were predicted based on the protein size (≤ 400 amino-acid residues) and the number of cysteine residues ( ⩾ 4) [68] . The prediction of transmembrane proteins and domain calling were described in the Supplementary Methods . Pectinolytic activity assays The pectinolytic activities of phytopathogenic fungi were evaluated using pectin plate assays as described previously with minor modifications [69] . Different fungi were grown on the pectin-containing media (1 l medium: 5.0 g pectin, 1.0 g yeast extract, 0.5 g glucose, 2.0 g KH 2 PO 4 , 1 g (NH 4 ) 2 SO 4 , 0.9 g Na 2 HPO 4 , trace of MnSO 4 , 15 g agar, pH 7.0). After colonies grew up to 4 cm in diameter, a 1% (w/v) CTAB solution was added to the plates. CTAB precipitates pectin present in the medium, resulting in opaque media where pectin was still present, and a transparent halo where pectin was broken down. The experiment was repeated three times. Growth profiles of U. virens on single carbon source Citrus pectin, glucose, xylan, cellulose and gum guar (all from Sigma) were used as single carbon source separately in agar medium, to evaluate the growth of different fungi. Inocula of U. virens and other fungi ( M. oryzae , R. solani , F. graminearum and C. fragariae ) were placed on these media and incubated at 28 °C with different cultivation times (21, 7, 5, 3 and 2 days, respectively). These tests were repeated three times, and the results were analysed to evaluate fungal mycelium growth, and graphed to visualize differences. Functional studies on putative effector proteins Putative effector genes (without signal peptide regions) of U. virens were amplified with the primer sets listed in Supplementary Table 31 . The PCR products were digested with the corresponding restriction emzymes and subcloned into pEDV [70] . Burkholderia glumae competent cells were prepared as described with minor modifications [43] . These pEDV constructs were transformed into B. glumae by electroporation. Leaves from 3-week-old Nicotiana benthamiana plants were infiltrated with B. glumae with different effector gene constructs or empty vector (OD600=0.4) using needleless syringes. Cell death symptoms were evaluated and photographed at 2–3 days after inoculation. How to cite this article : Zhang, Y. et al . Specific adaptation of Ustilaginoidea virens in occupying host florets revealed by comparative and functional genomics. Nat. Commun. 5:3849 doi: 10.1038/ncomms4849 (2014). Accession codes : The Whole-Genome Shotgun project for Ustilaginoidea virens has been deposited in DDBJ/EMBL/GenBank under the accession code JHTR00000000 .